Microwave spectroscopic observation of distinct electron solid phases in wide quantum wells In high magnetic fields, two-dimensional electron systems can form a number of phases in which interelectron repulsion plays the central role, since the kinetic energy is frozen out by Landau quantization. These phases include the well-known liquids of the fractional quantum Hall effect, as well as solid phases with broken spatial symmetry and crystalline order. Solids can occur at the low Landau-filling termination of the fractional quantum Hall effect series but also within integer quantum Hall effects. Here we present microwave spectroscopy studies of wide quantum wells that clearly reveal two distinct solid phases, hidden within what in d.c. transport would be the zero diagonal conductivity of an integer quantum-Hall-effect state. Explanation of these solids is not possible with the simple picture of a Wigner solid of ordinary (quasi) electrons or holes. Solid phases [1] , [2] , [3] , [4] , [5] , [6] , [7] , [8] of carriers are insulators, owing to pinning by disorder, and are not easily distinguishable from other types of insulators by standard d.c. transport measurements, but rather by a characteristic resonance, at frequency f pk in their microwave conductivity spectra [5] , [9] , [10] , [11] . These resonances are understood as pinning modes [5] , [11] in which pieces of the solid oscillate within the disorder potential, as diagrammed in Fig. 1a . Pinning modes have been found both near the low Landau filling ( v ) termination of the fractional quantum Hall effect (FQHE) series [5] , [10] and within the v ranges of integer quantum Hall effect (IQHE) plateaus [9] . In the weak pinning picture [12] , [13] , [14] , f pk increases when the shear modulus, C t , decreases, for example, by decreasing the density, n (ref. 15 ). The inverse relation of f pk and C t is because carriers associate more closely with minima in the disorder potential [12] , [13] , [14] . Consistent with this picture, in wells narrower than those studied here [9] , a solid within the IQHE range shows a monotonic decrease in f pk as v moves away from the quantizing filling, which increases the charge density of the solid. 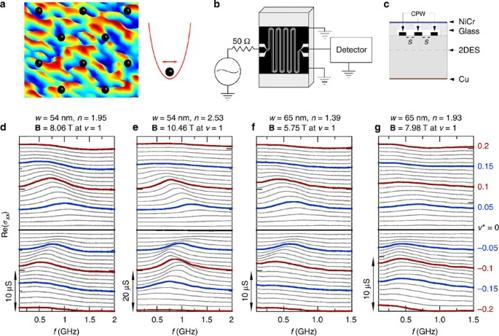Figure 1: Microwave spectroscopy of wide quantum wells. (a) Left: sketch of carriers (black) of an electron solid within the residual disorder potential, which is shown by colour (not to scale). Right: a piece (domain) of solid moves within a potential due to the disorder averaged over the domain, giving rise to the pinning mode studied here. (b) Schematic of the microwave set-up. The source and detector are at room temperature. A CPW transmission line is patterned on the top surface of the sample, with metal film of the CPW shown in black. (c) Side view of the sample (not to scale) shows the placement of the front and back gates and the metal film of the CPW. Slots of widthsseparate the centre conductor and ground planes of the CPW. (d,e) Spectra (diagonal conductivity Re(σxx) versus frequencyf) obtained from the 54 nm well withn=1.95 and 2.53, at severalv*=v−1, marked on the right axis ofg. Successive spectra are offset upward by 1 μS indand 2 μS ine. (f,g) Spectra for the 65 nm well atn=1.39 and 1.93 offset consecutively by 1 μS. For each spectrum the magnetic field,B, atv=1 is marked. Figure 1: Microwave spectroscopy of wide quantum wells. ( a ) Left: sketch of carriers (black) of an electron solid within the residual disorder potential, which is shown by colour (not to scale). Right: a piece (domain) of solid moves within a potential due to the disorder averaged over the domain, giving rise to the pinning mode studied here. ( b ) Schematic of the microwave set-up. The source and detector are at room temperature. A CPW transmission line is patterned on the top surface of the sample, with metal film of the CPW shown in black. ( c ) Side view of the sample (not to scale) shows the placement of the front and back gates and the metal film of the CPW. Slots of width s separate the centre conductor and ground planes of the CPW. ( d , e ) Spectra (diagonal conductivity Re( σ xx ) versus frequency f ) obtained from the 54 nm well with n =1.95 and 2.53, at several v *= v −1, marked on the right axis of g . Successive spectra are offset upward by 1 μS in d and 2 μS in e . ( f , g ) Spectra for the 65 nm well at n =1.39 and 1.93 offset consecutively by 1 μS. For each spectrum the magnetic field, B , at v =1 is marked. Full size image In the following, we report pinning modes whose f pk exhibits an upward step as v is decreased from 1, in contrast to the monotonic decrease in f pk that was seen in narrower wells. The phenomenon is seen in wide quantum wells (WQWs) [16] , [17] , [18] , [19] , [20] , in which the effective electron–electron interaction is softened at short range due to the large growth-direction extent of the wavefunction. A wider well, or a larger n , causes the step to move closer to v =1. We provide a natural interpretation, based on the sensitivity of f pk to the properties of the solid, that the step signals a transition between different solids. Sample details Our samples are from wafers containing GaAs quantum wells of widths w =54 and 65 nm. For both widths, the quantum wells were flanked on either side by undoped Al 0.24 Ga 0.76 As. Henceforth, in this paper all n will be in units of 10 11 cm −2 for brevity. The 54 nm well has depth of the two dimensional electron system (2DES) from the top d =430 nm, as-cooled n =2.42 and mobility μ =5.7 × 10 6 cm 2 V −1 s −1 at 300 mK. The 65 nm well has d =510 nm, as-cooled n =1.52, and μ =5.2 × 10 6 cm 2 V −1 s −1 at 300 mK. For the microwave measurement the sample temperature was 60 mK, measured in the mixing chamber of the dilution refrigerator. We verified that the samples were cooling along with the cryostat down to the reported temperature, by varying the cryostat temperature. d.c. data were taken at 20 mK. The data were taken with a growth-direction charge distribution that is approximately symmetric about the well centre with microwave data taken using the set-up in Fig. 1b,c (see Methods). Microwave spectroscopy The spectra, diagonal conductivity Re( σ xx ) versus frequency f , in Fig. 1d–g give an overview of the evolution of the resonance with Landau filling at different n for the two well widths. We present results in terms of v *= v −1, where | v *| is nearly proportional to the quasiparticle or hole density. In the smaller n states in Fig. 1d,f , and also for the larger n states in Fig. 1e,g with v *>0, resonances develop as in ref. 9 : as | v *| increases the resonance forms, develops maximal absorption around | v *|=0.08–0.10 and then fades away, all as f pk monotonically decreases with | v *|. The resonance development is different for the larger n states with v *<0. In Fig. 1e,g f pk decreases with decreasing v * but near v *~−0.08 begins to increase. Further decrease in v * results in an increase in f pk until v *~−0.12, below which f pk again decreases. f pk is extracted from the zero crossing of the imaginary conductivity, Im( σ xx ), versus f , as explained in Fig. 2 . Figure 3 shows plots of f pk versus v * at several n for the two WQWs. 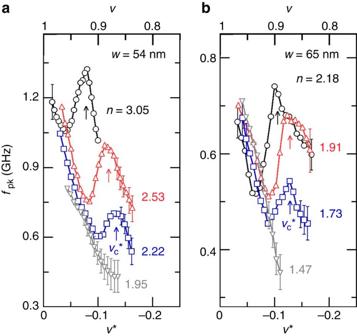Figure 3: Dependence of resonance peak frequency on filling factor. fpkversus partial Landau level fillingv* for the 54-nm (a) and 65-nm (b) wells at various carrier densities (n) as marked. Arrows mark*, thev* of the local maxima infpk. Data points without an attached error bar have estimated error, seeFig. 2for error discussion, infpkthat is smaller than ±5%. For the lowest n traces, f pk versus | v *| monotonically decreases, but for larger n a local minimum and maximum develop. 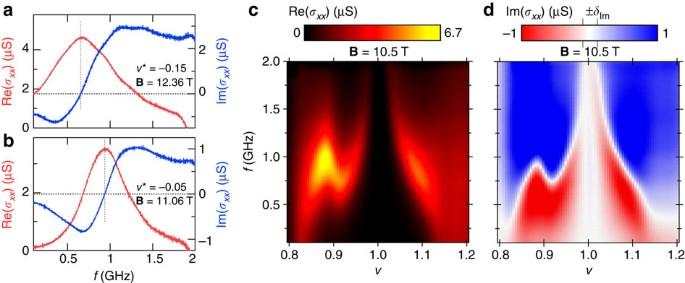The minimum and maximum move closer to v *=0 as n increases and are exhibited at lower n for the 65 nm sample. Figure 2: Resonance peak frequency extraction. (a,b) Real (left axis), and imaginary (right axis), parts of conductivityσxxversusfat two fixedv* and correspondingBas marked, obtained from the 54 nm well atn=2.53. Dotted vertical lines mark the zero crossing of Im(σxx) versusf, from whichfpkis determined. The error in Im(σxx), ±δIm=±0.08 μS, includes random noise and slower variation in Im(σxx) versusfdue to residual reflections near the sample mount. (c,d) Colour images in the (f,v) plane for Re(σxx) and Im(σxx), respectively, the magnetic field value forv=1 is marked on the figure. The colour scale indis set such that the centre of the white band is 0, and its extent in Im(σxx) is ±δIm. Thus, the white band in the image traces outfpkversusvand its height is ±δ(fpk). Figure 2: Resonance peak frequency extraction. ( a , b ) Real (left axis), and imaginary (right axis), parts of conductivity σ xx versus f at two fixed v * and corresponding B as marked, obtained from the 54 nm well at n =2.53. Dotted vertical lines mark the zero crossing of Im( σ xx ) versus f , from which f pk is determined. The error in Im( σ xx ), ± δ Im =±0.08 μS, includes random noise and slower variation in Im( σ xx ) versus f due to residual reflections near the sample mount. ( c , d ) Colour images in the ( f , v ) plane for Re( σ xx ) and Im( σ xx ), respectively, the magnetic field value for v =1 is marked on the figure. The colour scale in d is set such that the centre of the white band is 0, and its extent in Im( σ xx ) is ± δ Im . Thus, the white band in the image traces out f pk versus v and its height is ± δ ( f pk ). Full size image Figure 3: Dependence of resonance peak frequency on filling factor. f pk versus partial Landau level filling v * for the 54-nm ( a ) and 65-nm ( b ) wells at various carrier densities ( n ) as marked. Arrows mark *, the v * of the local maxima in f pk . Data points without an attached error bar have estimated error, see Fig. 2 for error discussion, in f pk that is smaller than ±5%. Full size image We interpret the results in terms of a transition between two distinct solids. Each of the solids exhibits a single pinning mode, and the step in pinning mode frequency, f pk , marks the change from one type of electron solid to the other. At the lowest n for both samples, f pk monotonically decreases with | v *|. At larger n , the f pk versus v * curves can be divided into two regions. In the smaller | v *| regions (closer to v =1), f pk versus v * tends towards the lowest n curve, while in the larger | v *| regions, to the right of the local maximum in Fig. 3 , f pk versus v * is enhanced relative to the lowest n curve. We take the enhanced pinning mode frequency f pk as a characteristic of a solid, which we call S2. It is distinct from S1, which is the only solid seen in the lowest n states of the samples, and which in the larger n states is closer to v *=0. With increasing n , the transition from S2 to S1 moves closer to v *=0, and the transition appears at lower n in the larger w sample. For larger n than those shown in Fig. 3 , the step to enhanced f pk as | v *| increases can be visible for v *>0 also, as is shown in Supplementary Fig. 1 . The transition thus appears to occur on both sides of v =1; therefore, S2 is favoured by larger n , w and | v *|. Longitudinal transport measurements We also perform d.c. transport measurements on the same wafers and find that the solid–solid transition picture can underlie features found earlier [17] in d.c. transport. WQWs were recently found [17] to exhibit v ranges that are not contiguous with the IQHE minimum centred at v =1, but still have Hall resistance quantized at h / e 2 and vanishing d.c. longitudinal resistance ( R xx ). These regions are called re-entrant integer quantum Hall effects (RIQHEs) [21] and are due to insulating phases of the partially filled Landau level. At sufficiently high n , the RIQHEs appear near v =4/5 (ref. 17 ). The RIQHE range extends towards v =1 as n is increased by gating, and eventually merges with the main IQHE plateau. The RIQHE was ascribed [17] to a Wigner solid, which can be favoured [22] over FQHE liquids in WQWs, owing to the softening of the effective electron–electron interaction at short range. The RIQHE sets in for w / l B ≳ 4, where l B =( h / eB ) 1/2 is the magnetic length. 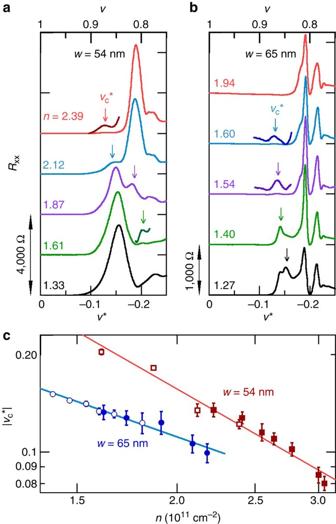Figure 4: Longitudinal transport, comparison with microwave resonance spectroscopy. (a,b) Longitudinal resistance versus partial Landau level fillingv* measured for the 54 nm (a) and the 65 nm (b) wells at different densitiesnas marked, vertically offset for clarity. Arrows mark*, the critical partial filling factor. WhereRxxis small, the trace in the region of* are duplicated and magnified 10 times for clarity. (c) |*| versusnon a log–log scale deduced from d.c. transport measurements (open symbols) and microwave spectra (solid symbols) for the 54 nm (squares) and 65 nm (circles). Error bars are based on the width of*. Power law fits of the form*∝n−αare also shown on the plot, whereα=1.35±0.1 and 0.87±0.07 for the 54 and 65 nm wells, respectively. Figure 4a,b shows plots of R xx versus v * for the 54 and 65 nm wells at several n . Just closer to v *=0 than the minimum due to the RIQHE, the R xx traces have peaks, both in ref. 17 and in Fig. 4a,b , which are denoted with arrows. With increasing n , the v * of the peak increases as the RIQHE minimum deepens. At the highest n , the peak vanishes as the RIQHE minimum merges with the main IQHE minimum. This peak in R xx could be produced by domain-wall conduction at a phase transition [17] , [23] . Figure 4: Longitudinal transport, comparison with microwave resonance spectroscopy. ( a , b ) Longitudinal resistance versus partial Landau level filling v * measured for the 54 nm ( a ) and the 65 nm ( b ) wells at different densities n as marked, vertically offset for clarity. Arrows mark *, the critical partial filling factor. Where R xx is small, the trace in the region of * are duplicated and magnified 10 times for clarity. ( c ) | *| versus n on a log–log scale deduced from d.c. transport measurements (open symbols) and microwave spectra (solid symbols) for the 54 nm (squares) and 65 nm (circles). Error bars are based on the width of *. Power law fits of the form * ∝ n − α are also shown on the plot, where α =1.35±0.1 and 0.87±0.07 for the 54 and 65 nm wells, respectively. Full size image Microwave spectroscopy and d.c. transport comparison To directly compare microwave and d.c. measurements, we define the critical filling * as that of the local maximum in the f pk versus v * measurements and that of the n -dependent peak in R xx versus v *, marked by arrows in Figs 3 and 4 . This results in continuous plots of * versus n , as shown in Fig. 4c , so that S2 can be identified with the d.c. RIQHE. The v * ranges of * versus n obtained from microwave and d.c. overlap at intermediate n and are remarkably consistent over the entire n range. Resonances for S2 set in at larger n than required to see the d.c. transport RIQHE, and can be seen at smaller | v *|. When the RIQHE merges with the IQHE the R xx peak at * is no longer visible, even when the transition is clearly visible in f pk . Pinning modes are not visible in the RIQHE ranges at larger | v *|, possibly because uncondensed carriers are present, which dampen the resonance. Chen et al. [10] reported evolution of the pinning mode with v below the termination of the FQHE series, in quantum wells with w =50 and 65 nm, but with much lower n ( ≃ 1 and 0.5, respectively) than those studied here. For 0.12< v <0.18, the spectra appeared irregular with multiple peaks, although well-defined peaks appeared above and below that range. In ref. 10 that v range was the same in each sample, and for v ≳ 0.18, the resonance was wave vector ( q )-dependent. The q dependence was found by comparing transmission lines of different slot width, s , q ~π/ s (see Methods). Checking for q dependence in the present 54 nm WQW sample using s =80 μm we found none, with excellent agreement between the s =80 μm f pk versus v * and the s =30 μm data shown in Fig. 3a . Since a pinning mode is identified with electron solids, an enhanced f pk similar to that of S2 relative to S1 is because of better ‘contact’ between the carriers of the solid and the disorder, increasing the effective pinning. This can be because of a smaller C t in S2 than in S1, as mentioned above, but the disorder contact can also be increased by a change in the charge distribution of each carrier in the lattice or in the lattice type (for example, from one-component to two-component). Theories [7] , [24] , [25] , [26] have considered crystals of composite fermions [27] , which are categorized by the number, 2p, of vortices bound to a carrier. Theory predicts a series of distinct composite fermion Wigner solid ( 2p CFWS) phases with 2p increasing as v decreases [7] , [24] . The transition from 2p=2–4 occurs as v goes from 1/5 to 1/6. Although 4 C t is predicted to soften near the transition, well within the 4 CFWS it is calculated to be a factor of ~2 larger than 2 C t and would result in a lower f pk in the 4 CFWS. Identifying S2 as a 2 CFWS and S1 as a 4 CFWS would be consistent with the shear moduli predicted by ref. 7 . However, ref. 7 predicts little sensitivity of the phase diagram to w , but we do observe dependence of * on w and n . Are there other possible interpretations for the two solids? A two-component bilayer Wigner solid can exist under certain conditions in a WQW [18] , [19] , particularly if the sub-band gap, Δ, is small enough relative to the Coulomb energy, E c . Such a two-component Wigner solid could have increased disorder and f pk because of charge being pushed closer to the interfaces [12] and would be favoured by larger | v *|, giving smaller carrier spacing, and by larger w . For the 54 nm well with typical v c =−0.1, n =2.8, we find from simulations [16] , [18] that Δ ~16 K, which according to ref. 28 is about three times too large for a two-component lattice to form. A composite fermion ground-state spin transition [29] , [30] is also unlikely to explain the observed phenomena. The composite fermion spin-Landau levels only cross above the Fermi level [30] . Although skyrmion solid formation has been reported [31] from pinning modes near v =1, at the larger * studied here large quasihole density would suppress skyrmion effects [32] . In summary, near v =1 in WQWs, we have found a change in f pk that is naturally interpreted as signature of a transition between two different solids. S2, which exists at larger | v *|, larger n and larger w , has enhanced f pk relative to the other phase. While the origin of the transition remains unclear, the possibilities, particularly of a transition in CFWS vortex number, are of fundamental importance. Charge distribution For d.c. measurements, the symmetry of the charge distribution about the well centre was maintained using the Fourier transform of R xx versus B in the Shubnikov–de Haas regime to minimize the gap, Δ, between the lowest and first excited sub-bands [16] , [20] . For the microwave measurements, balance of the change between front and back halves of the well was maintained by biasing front and back gates such that individually each would change the carrier density by equal amounts. Microwave spectroscopy technique Our microwave spectroscopy [2] technique [9] , [10] , [31] uses a coplanar waveguide (CPW) on the surface of a sample. A NiCr front gate was deposited on glass that was etched to space it from the CPW by ~10 μm. A schematic diagram of the microwave measurement technique is shown in the left panel of Fig. 1b and side view of the sample is shown in Fig. 1c . The microwave electronics, consisting of a pre-amplifier, network analyser (Agilent E5071 C) and attenuators, was entirely located at room temperature. Semi-rigid coaxial cables, including both copper and superconducting types, were used within the cryostat to connect the sample to room-temperature ports at the cryostat top. The connections are carefully optimized to minimize reflections, and the incident power on the sample fluctuates only ~10% because of standing waves on the coaxial cables. The effects of these standing waves, and of the frequency-dependent loss of the cables, were largely removed by taking the ratio t / t 0 , where t was the amplitude at the receiver and t 0 is the amplitude for v =1. We calculate the diagonal conductivity as σ xx ( f )=( s / lZ 0 ) ln( t/t 0 ), where s =30 μm is the distance between the centre conductor and ground plane, l =28 mm is the length of the CPW and Z 0 =50 Ω is the characteristic impedance without the 2DES. Hence, σ xx ( f ) is the difference between the conductivity and that for v =1; just at v =1 the conductivity is vanishing at low temperature. The microwave measurements were carried out in the low-power limit, where the measurement is not sensitive to the excitation power. Longitudinal transport measurements For d.c. transport measurements, no transmission line was used; measurements were performed in a van der Pauw geometry using standard ( ≃ 30 Hz) lock-in technique, with front and back gates both deposited directly on the sample surfaces. How to cite this article: Hatke, A. T. et al. Microwave spectroscopic observation of distinct electron solid phases in wide quantum wells. Nat. Commun. 5:4154 doi: 10.1038/ncomms5154 (2014).